Electrically tunable multiple Dirac cones in thin films of the (LaO)2(SbSe2)2family of materials Two-dimensional Dirac physics has aroused great interests in condensed matter physics ever since the discovery of graphene and topological insulators. The ability to control the properties of Dirac cones, such as bandgap and Fermi velocity, is essential for various new phenomena and the next-generation electronic devices. On the basis of first-principles calculations and an analytical effective model, we propose a new Dirac system with eight Dirac cones in thin films of the (LaO) 2 (SbSe 2 ) 2 family of materials, which has the advantage in its tunability: the existence of gapless Dirac cones, their positions, Fermi velocities and anisotropy all can be controlled by an experimentally feasible electric field. We identify layer-dependent spin texture induced by spin–orbit coupling as the underlying physical reason for electrical tunability of this system. Furthermore, the electrically tunable quantum anomalous Hall effect with a high Chern number can be realized by introducing magnetization into this system. Unlike the usual materials with parabolic energy dispersion described by the non-relativistic Schrodinger equation, graphene [1] provides the first example in condensed matter physics with low-energy effective physics described by the relativistic Dirac equation with linear energy dispersion. Later, it was realized that two-dimensional Dirac type of dispersion also appears for the surface states of three-dimensional topological insulators [2] , [3] , of which spin is resolved and locked to the momentum, forming a spin texture in the surface Brillouin zone. Dirac Hamiltonians with or without mass also exist in the low-energy physics of several other families of materials, including topological crystalline insulators (such as SnTe (refs 4 , 5 , 6 )), group-VI dichalcogenides (such as MoS 2 (refs 7 , 8 , 9 , 10 , 11 )), SrMnBi 2 (ref. 12 ), d -wave cuprate superconductors [13] , and three-dimensional Dirac semimetals (such as Na 3 Bi (ref. 14 ), Cd 3 As 2 (refs 15 , 16 )). Owing to the similar energy dispersion, all these materials share some common and unique physical properties, thus dubbed Dirac materials [17] , which are believed to have potential applications in high performance nanoelectronics [1] , spintronics and quantum computation [2] , [3] . In these existing Dirac materials, the properties of Dirac cones, such as the position and Fermi velocity, are usually determined by intrinsic properties of the materials, such as crystal structures and spin–orbit coupling (SOC), and thus they are difficult to control experimentally. For example, pristine graphene [1] does not have a bandgap, so for the potential application in transistors, one needs bilayer graphene [18] , [19] , of which the energy dispersion becomes parabolic. Therefore, it is desirable to have Dirac materials with the properties of Dirac cones tunable by external experimental conditions. In this paper, we propose a new family of Dirac materials, including ( R O) 2 ( MX 2 ) 2 (refs 20 , 21 , 22 , 23 ) and ( Ae F) 2 ( MX 2 ) 2 (refs 24 , 25 , 26 ) ( R =rare earth, Ae =Sr or Ba, M =Sb or Bi, X =S, Se or Te, O=oxygen and F=fluorine). The multiple Dirac cones and the electrical tunability of Dirac physics in this system allow us to obtain the quantum anomalous Hall (QAH) effect with higher Chern number, which can be controlled by a gate voltage. Electrically tunable Dirac cones To illustrate crystal structures of this family of materials, we may take (LaO) 2 (SbSe 2 ) 2 as an example, which possesses the tetragonal ZrCuSiAs-type structure [27] with space group P 4/ nmm . As shown in Fig. 1a , (LaO) 2 (SbSe 2 ) 2 has a triple-layer (TL) structure with one (LaO) 2 layer sandwiched by two SbSe 2 layer in one unit cell. The (LaO) 2 layer is similar to that in LaOFeAs (ref. 28 ), formed by a square lattice of O atoms, coordinated tetrahedrally with four neighbouring La atoms. However, the SbSe 2 layer has a different structure from the FeAs layer. For one SbSe 2 layer, the Sb 1 atom and Se 2 atom form a distorted checkerboard lattice while the Se 1 atom lies between (LaO) 2 layer and the checkerboard SbSe layer. Each Sb atom can be viewed to have a distorted octahedral coordination with six Se atoms. Strong ionic bonding is formed between the central (LaO) 2 layer and two adjacent SbSe 2 layers within one unit cell while the chemical bonding between two adjacent SbSe 2 layers in neighbouring unit cells is much weaker, dominated by van der Waals interaction [29] . The primitive lattice vectors are shown in Fig. 1a , denoted as x, y, z. The lattice constant is denoted as a along the x and y directions and c along the z direction. The space group P 4/ nmm is non-symmorphic and possess a glide operation which consists of a reflection in the x – y plane, , followed by a non-primitive translation . The system has inversion symmetry with the inversion centre located at the centre of two nonequivalent O atoms. In addition, there is a mirror symmetry along both the x and y directions, denoted as and . 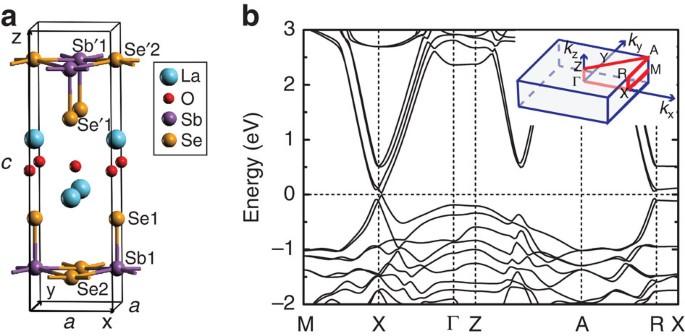Figure 1: Crystal structure and bulk band dispersion. (a) Primitive cell of (LaO)2(SbSe2)2crystal structure. (b) Band structure of (LaO)2(SbSe2)2along the high symmetric lines that are depicted by red lines in bulk Brillouin zone (the inset). Figure 1: Crystal structure and bulk band dispersion. ( a ) Primitive cell of (LaO) 2 (SbSe 2 ) 2 crystal structure. ( b ) Band structure of (LaO) 2 (SbSe 2 ) 2 along the high symmetric lines that are depicted by red lines in bulk Brillouin zone (the inset). Full size image Based on the density-functional theory, we calculate the electronic band structure of (LaO) 2 (SbSe 2 ) 2 , which is found to be a narrow gap semiconductor with the bandgap near the X and Y points in the Brillouin zone, as shown in Fig. 1b . Both conduction and valence bands are fourfold degenerate at X and split into two doubly degenerate states along the Γ-X line. An anti-crossing occurs between the conduction and valence bands along the Γ-X line, resulting in a bandgap around 20 meV. In addition, the band structure is found to be non-dispersive along the line Γ-Z and R-X, indicating that adjacent TLs are weakly coupled and the system is essentially two dimensional. Therefore, we will study a film configuration with one TL of (LaO) 2 (SbSe 2 ) 2 . It has recently been shown that a TL film is stable for one material (LaO) 2 (BiS 2 ) 2 in this family [29] . The configuration of a TL film is shown schematically in Fig. 2a , with front and back gate voltages V g , which provide an electric field E ex or an effective asymmetric potential e U on the thin film. 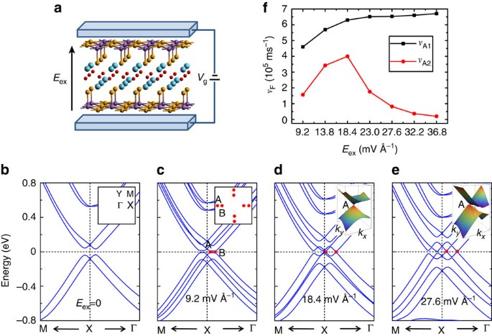Figure 2: Electric tunability of Dirac cones. (a) Schematic plot of a TL film of (LaO)2(SbSe2)2with a gate voltageVgor an electric fieldEex. (b–e) Band dispersions of a TL film near X under the electric fieldsEex=0, 9.2, 18.4, 27.6 mV Å−1, respectively. The inset ofbshows the Brillouin zone and inset ofcshows the positions of the gapless points in the Brillouin zone. The red dots depict gapless points. The insets ofdandeshow Dirac cones at the red dots close to the X point from the first-principles calculations. The plot range is,, −0.02 eV≤E≤0.02 eV ford, and,, −0.06 eV≤E≤0.06 eV fore. (f) The Fermi velocity is shown as a function of the electric fieldEex.vA1(vA2) indicates the velocity of Dirac cone A along the direction ofkx(ky). Figure 2b–e show band dispersion under the electric field E ex =0, 9.2, 18.4, 27.6 mV Å −1 , respectively. With increasing electric fields, the double degeneracy along the Γ-X line is split, and the bandgap is reduced and closed around E ex =9.2 mV Å −1 . From Fig. 2c–e , one can clearly see that for the electric field E ex ⩾ 9.2 mV Å −1 , the bandgap will re-open along the X-M line while it remains gapless along the Γ-X line. There are totally eight gapless points in the whole Brillouin zone, four around X and four around Y, and their positions in the Brillouin zone are indicated by red dots in the inset of Fig. 2c . Each gapless point forms a Dirac cone with linear dispersion, as shown in the insets of Fig. 2d,e . These eight Dirac cones can be classified into two sets: four equivalent Dirac cones (A) are close to X or Y while the other four (B) are away from these two momenta. We emphasize that all the Dirac cones here are spin resolved, different from that in graphene but similar to the case of topological insulators. Strikingly, the properties of Dirac cones, such as their positions, velocities and anisotropy, are tunable with electric fields. For example, the velocity of Dirac fermions around X is shown as a function of the electric field E ex in Fig. 2f , which can be tuned in the range (4.6 ∼ 6.7) × 10 5 m s −1 along the k x direction and (0.2 ∼ 4.0) × 10 5 m s −1 perpendicular to k x with the experimentally feasible electric field [30] , [31] (the corresponding voltage drops between the two checkerboard SbSe layers are in the range 0 ∼ 400 mV (see Supplementary Fig. 1 and Supplementary Note 1 for the relationship between the electric field and the atomic layer energy splitting)). We notice that the velocity of linear dispersion has a small anisotropy for E ex <18.4 mV Å −1 , while the velocity anisotropy increases rapidly when E ex ⩾ 18.4 mV Å −1 , as clearly shown in the insets of Fig. 2d,e . At the electric field E ex =36.8 mV Å −1 , the velocity along the Γ-X direction is around 7 × 10 5 m s −1 , about four times smaller than that in graphene, while that perpendicular to the Γ-X direction is one order smaller (2 × 10 4 m s −1 ). To understand the existence and tunability of Dirac cones, we will next develop a low-energy effective model for this system. Figure 2: Electric tunability of Dirac cones. ( a ) Schematic plot of a TL film of (LaO) 2 (SbSe 2 ) 2 with a gate voltage V g or an electric field E ex . ( b – e ) Band dispersions of a TL film near X under the electric fields E ex =0, 9.2, 18.4, 27.6 mV Å −1 , respectively. The inset of b shows the Brillouin zone and inset of c shows the positions of the gapless points in the Brillouin zone. The red dots depict gapless points. The insets of d and e show Dirac cones at the red dots close to the X point from the first-principles calculations. The plot range is , , −0.02 eV≤ E ≤0.02 eV for d , and , , −0.06 eV≤ E ≤0.06 eV for e . ( f ) The Fermi velocity is shown as a function of the electric field E ex . v A1 ( v A2 ) indicates the velocity of Dirac cone A along the direction of k x ( k y ). Full size image Low-energy effective model To develop a theoretical model, we first check the orbital natures of conduction and valence bands. The band structure with different atomic projections is shown in Fig. 3a,b . The orbitals of La and O atoms lie far away from the Fermi energy due to the strong electron negativity and affinity. The outmost shells for both Sb (5 s 2 5 p 3 ) and Se (4 s 2 4 p 4 ) are p orbitals. The Se 1 and atoms are close to the (LaO) 2 layer and form strong bonds, which push their energy levels away from the Fermi energy. Thus, the bands near the Fermi energy are dominated by the p orbitals of Sb 1 and Se 2 atoms in the SbSe checkerboard layers. Therefore, we focus on the bilayer SbSe checkerboard lattice and develop an atomic tight-binding model on this lattice with three p orbitals on each site. The details of lattice structures ( Supplementary Fig. 2 ) and the form of tight-binding model are described in Supplementary Note 2 . By carefully choosing parameters, we can qualitatively reproduce energy dispersions near X (or Y) and four Dirac cones emerge along the Γ-X line after turning on an asymmetric potential between two layers, as shown in Fig. 3c,d , Supplementary Fig. 3 and Supplementary Note 3 . 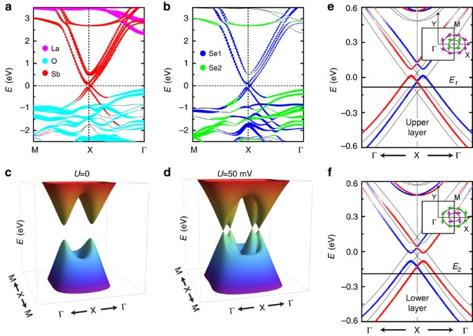Figure 3: Atomic orbital and spin nature of band structure. (a,b) Band structures with different atomic projections. The atomic characters La, O, Sb, Se1and Se2are indicated by magenta, cyan, red, green and blue, respectively. (c,d) Band structure around X from tight-binding model, withU=0 incandU=50 mV ind. (e,f) Theab initiocalculations of spin-resolved bands with the upper (ine) and lower (inf) SbSe checkerboard layer projection under the electric fieldEex=9.2 mV Å−1. The red and blue denote the states of spin up and spin down, which are polarized along theydirection. The two insets schematically reveal the spin textures under the iso-energetic contours with the energyE1andE2, respectively. Figure 3: Atomic orbital and spin nature of band structure. ( a , b ) Band structures with different atomic projections. The atomic characters La, O, Sb, Se 1 and Se 2 are indicated by magenta, cyan, red, green and blue, respectively. ( c , d ) Band structure around X from tight-binding model, with U =0 in c and U =50 mV in d . ( e , f ) The ab initio calculations of spin-resolved bands with the upper (in e ) and lower (in f ) SbSe checkerboard layer projection under the electric field E ex =9.2 mV Å −1 . The red and blue denote the states of spin up and spin down, which are polarized along the y direction. The two insets schematically reveal the spin textures under the iso-energetic contours with the energy E 1 and E 2 , respectively. Full size image Below, we will focus on the effective theory around X (or Y). We find that the conduction band minimum and valence band maximum are dominated by p x ( p y ) orbitals of Se and Sb atoms around the X (Y) point. This orbital nature is confirmed by the ab initio calculation, as shown in Supplementary Fig. 4 of Supplementary Note 4 . As described above, both conduction and valence bands have fourfold degeneracy at X, which originates from two spin states and two checkerboard SbSe layers. Therefore, we can construct a four band effective model around X on the basis | p x , σ , ξ μ 〉 for the conduction and valence bands respectively, where σ = z , z denotes spin, ξ =c,v denotes conduction band and valence band and μ =± denotes the upper and lower layer. We choose the spin axis along the z direction. It should be emphasized that there is a strong hybridization between Se and Sb atoms for both the conduction and valence bands near the bandgap. Thus, we use ξ =c,v instead of Sb, Se to denote the basis. Using the Lowdin perturbation method [32] , we find the effective Hamiltonian takes the form around X up to the second order in k for the conduction or valence band, where , the Pauli matrices denote layer index and denote spin index. d iξ and f iξ are material dependent parameters, and can be extracted from perturbation procedure. In the Hamiltonian (1), the first term is not important. The second term is a spin-independent term, describing the hybridization between two layers. The third and fourth terms depend on spin and originate from the third order perturbation combining the interlayer hopping and SOC (see Supplementary Note 5 ). We notice that these two terms take the familiar form of the Rashba type of Hamiltonian while the additional dependence indicates that the spin splitting is opposite for two layers. This layer-dependent Rashba term is the origin of the layer-dependent spin texture described below. The last term describes the asymmetric potential e U induced by electric fields. We next look at the symmetry properties of Hamiltonian (1). The present system has time reversal symmetry and the space group symmetry P 4/ nmm . The wavevector group of P 4/ nmm at X contains glide symmetry , mirror symmetry and inversion symmetry . The effective Hamiltonian (1) can be derived from symmetry principles based on the above symmetries, as shown in Supplementary Note 6 and Supplementary Table 1 . We find that the fourfold degeneracy at X can be determined from three symmetry operations , and . On the basis | σ , μ 〉 of the effective Hamiltonian (we neglect p x and ξ for short), the representation of symmetry operators is given by , and for conduction (valence) bands, where K is complex conjugate. Since [ m y , H ξ ]=0 at X, we may choose eigen states with definite mirror parity of . Four eigen states can be written as , which satisfy . Here y and y correspond to up and down spin along the y direction. Now let us consider how and act on these four states | ψ μ , σ y 〉 . Both and change spin up y to spin down y . However, the obtained states operated by or are different since the layer index is preserved by but changed by . In addition, the combination of and leads to the state with the same spin but different layer indices. Thus, these four eigen states can be related to each other by , and , so they must be degenerate at X. In general, the fourfold degeneracy at the X (Y) point is a direct consequence of the combination of time reversal symmetry and the anti-commutation relation between and . After understanding the degeneracy at X, we next consider the states away from X along the Γ-X line ( k x 0, k y =0 in Hamiltonian (1)). In Fig. 2b , one can see that fourfold degenerate states are split into two doubly degenerate states. According to Hamiltonian (1), both the hybridization term ( f 1 ξ term) and the SOC term ( f 2 ξ and f 3 ξ terms) can contribute to this splitting. The remaining double degeneracy at a finite k x comes from the combined symmetry (Kramers’ doublet due to both the time reversal symmetry and inversion symmetry). Alternatively, we can also understand it from the combination of and . We can still choose two degenerate eigen states to have definite mirror parity, denoted as m y | ψ y ( y ) ( k x )〉=+ i (− i )| ψ y ( y ) ( k x )〉. It should be emphasized that the states | ψ y ( y ) ( k x )〉 should be a linear combination of the basis in different layers. | ψ y ( k x )〉 and | ψ y ( k x )〉 are still related to each other by , which will also change the layer index. This means that if | ψ y ( k x )〉 mainly stays at the upper layer, | ψ y ( k x )〉 must be at the lower layer. Thus, spin and layer indices are related to each other, leading to the layer dependence of spin textures in this system. To show it more explicitly, we calculate spin polarization at a given momentum k for different layers based on the effective model (1). As an example, we may consider spin texture of two degenerate eigen states ( α =1,2) with eigen energy , which is given by where the layer-dependent spin operator is defined as with i = x , y , z . From Equation (2), we indeed find opposite spin textures for different layers once the parameter f 2 ξ or f 3 ξ , originating from SOC, is non-zero. Now let us turn on the asymmetric potential e U between two layers. Since spin states are locked to the layer indices, two spin states with opposite layer indices will be split accordingly. This picture has been used to explain the giant Rashba spin splitting in (LaO) 2 (BiS 2 ) 2 in the early study [29] , [33] . In our case, we need to consider spin splitting for both conduction and valence bands. It is found that the parameters f 2c and f 2v have opposite signs ( f 2c >0 and f 2v <0) while f 3c and f 3v have the same sign ( f 3c , f 3v <0), leading to different spin textures for the conduction and valence bands. From the Supplementary Note 7 and Supplementary Fig. 5 , for the case with U >0, k x >0 and k y =0, the lowest conduction band carries spin up at the lower layer while the highest valence band is dominated by the states with spin down at the upper layer. Since these two states have opposite spin, as well as opposite mirror parities of , there is no coupling between them. Thus, the Dirac cones due to the crossing points between the conduction and valence bands along the Γ-X line are protected by mirror symmetry. From the above analysis, we can see that the layer-dependent spin texture is the underlying physical reason for the existence and tunability of Dirac cones. To further confirm our physical picture, we perform the first-principles calculations of layer-dependent spin texture in this system, as shown in Fig. 3e,f . Figure 3e (f) is the spin-resolved band projecting on the upper (lower) SbSe checkerboard layer at the electric field E ex =9.2 mV Å −1 . The opposite spin textures for the upper and lower SbSe layer are shown in the insets of Fig. 3e,f , respectively. Electrically tunable QAH effect When gapless Dirac cones are gapped by magnetization, quantized Hall conductance is possible to arise even at a zero magnetic field and without Landau levels. This phenomenon is known as the QAH effect [34] , [35] , [36] , [37] , [38] , which was recently observed in Cr or V doped (Bi,Sb) 2 Te 3 films experimentally with the quantized Hall conductance (Chern number 1; refs 39 , 40 ). Multiple Dirac cones systems allow for the realization of the QAH effect with a larger Chern number, which was first proposed in graphene systems [41] , as well as other systems, including magnetically doped (Bi,Sb) 2 Te 3 films [42] and SnTe systems [43] . Here we will consider the exchange coupling of magnetic moments and predict the QAH effect with a high Chern number in magnetically doped (LaO) 2 (SbSe 2 ) 2 , which can be controlled by an external electric field. To theoretically study how exchange coupling affects our system, we construct a more realistic tight-binding model using the maximum localized Wannier function method [44] , [45] , and then introduce exchange coupling phenomenologically. This method has been widely adopted to study the QAH effect in magnetically doped topological insulators [38] , [46] . We start from the case with an asymmetric potential e U =100 meV and no magnetization, in which eight Dirac cones exist in the whole Brillouin zone. The results obtained from the Wannier function method is consistent with the direct calculation from the first-principles methods. The exchange coupling is introduced into the calculation by the phenomenological Kondo-type of Hamiltonian H ex = J ex s · M , where J ex is the exchange coupling constant, s denotes electron spin and M is the average magnetization of the system. The Dirac cones are gapped by turning on magnetization (see Supplementary Fig. 6 in Supplementary Note 8 ). It is well-known that each gapped 2D Dirac cone (massive Dirac Hamiltonian) contributes half quantized Hall conductance . Thus, the total Hall conductance is determined by the sign of the Hall conductance contribution from different Dirac cones. It turns out that all massive Dirac Hamiltonians take the same sign, leading to the total Hall conductance for the whole system. To see this more explicitly, we directly calculate edge states of the whole system in a ribbon configuration and plot the local density of states at one edge along the x direction. We take (SrF) 2 (SbSe 2 ) 2 as an example owing to its large electric tunability. Similar results can also be obtained for other systems in this class of materials, as shown in the Supplementary Note 8 and Supplementary Fig. 7 . As shown in Fig. 4a,b , there are in total four chiral edge states propagating along the same direction, with two appearing near the point and the other two near the point, where and are the projection of Γ and X into the one-dimensional edge. Therefore, the edge state picture is consistent with the analysis of bulk Dirac cones, revealing that the QAH state with the Hall conductance can be realized in this system. 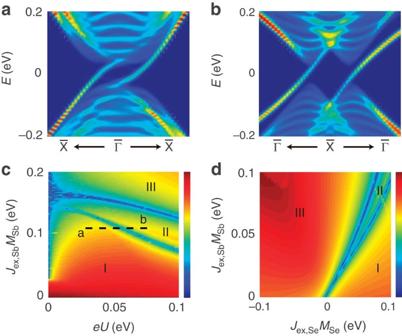Figure 4: Electrically tunable QAH effect. The local density of states at one edge of a ribbon of (SrF)2(SbSe2)2film near thepoint inaand near thepoint inbforeU=0.1 eV andJex,SeMSe=−Jex,SbMSb=0.05 eV. Two chiral edges are found nearwhile the other two near. The bulk bandgap is plotted as a function ofJex,SbMSbandeUincforJex,SeMSe=0.1 eV, while it is shown as a function ofJex,SbMSbandJex,SeMSeindforeU=0.05 eV. Here the gaps are plot in logarithmic scale and blue colour is for gap closing. We find two gapless lines (blue lines) divide the phase diagram into three regimes I, II and III with Hall conductance, 0 and, respectively. By tuning the electric field the states can move along the dashed line from a to b. Figure 4: Electrically tunable QAH effect. The local density of states at one edge of a ribbon of (SrF) 2 (SbSe 2 ) 2 film near the point in a and near the point in b for eU =0.1 eV and J ex,Se M Se =− J ex,Sb M Sb =0.05 eV. Two chiral edges are found near while the other two near . The bulk bandgap is plotted as a function of J ex,Sb M Sb and eU in c for J ex,Se M Se =0.1 eV, while it is shown as a function of J ex,Sb M Sb and J ex,Se M Se in d for eU =0.05 eV. Here the gaps are plot in logarithmic scale and blue colour is for gap closing. We find two gapless lines (blue lines) divide the phase diagram into three regimes I, II and III with Hall conductance , 0 and , respectively. By tuning the electric field the states can move along the dashed line from a to b. Full size image Figure 4c,d show bulk bandgap as a function of magnetization ( J ex,Sb M z ,Sb and J ex,Se M z ,Se ) and asymmetric potential e U . Since a topological phase cannot be changed when the bulk bandgap remains open, the phase diagram can be determined by tracking the gap closing lines [37] . Two gapless lines are found in Fig. 4c , indicating two topological phase transitions. For each metallic line, four equivalent Dirac cones (Dirac cones A or B in the inset of Fig. 2c ) reverse their bandgap, leading to the change of Hall conductance by . Therefore, we can determine the Hall conductance in each regime, as dictated by the regimes I, II and III in Fig. 4c with Hall conductance , 0 and , respectively. We emphasize that along the dashed line a − b in Fig. 4c , a topological phase transition from the Hall conductance to 0 can occur by tuning only electric fields and fixing magnetization. This again reflects the electrical tunability of Dirac physics in this system, as discussed in the above section. The physics discussed above for (LaO) 2 (SbSe 2 ) 2 can also be applied to other materials in this family. Since all low-energy physics occurs in the SbSe 2 layer, the (LaO) 2 layer can also be replaced by other ( R O) 2 layer where R is a rare earth atom. As shown in Supplementary Note 4 and Supplementary Fig. 8 , the SbSe 2 layer can also be replaced by other Sb X 2 layers ( X =Te, S). For Bi X 2 ( X =S,Te,Se) (refs 47 , 48 ), an indirect bandgap occurs, ranging from 70 to 300 meV, and is not suitable for electric control. In addition, the (LaO) 2 layer can also be replaced by ( Ae F) 2 where Ae =Sr, Ba (refs 24 , 25 , 26 ). Experimentally, bulk (LaO) 2 (SbSe 2 ) 2 and ( Ae F) 2 (SbSe 2 ) 2 have been fabricated by the high-temperature ceramic method [20] , [24] . As shown in Supplementary Note 9 and Supplementary Fig. 9 , the binding energy between the TLs for (LaO) 2 (SbSe 2 ) 2 is about 7.3 meV Å −2 without van der Waals correction and 30.7 eV Å −2 with van der Waals correction, comparable to that of MoS 2 ( ∼ 20 meV Å −2 ) (ref. 49 ). The exfoliation of TL (LaO) 2 (SbSe 2 ) 2 is expected to be feasible in experiments. For the case of multiple TLs, Dirac cones also exist but may be buried in other bulk bands, as shown in the Supplementary Note 10 and Supplementary Fig. 10 . The effect of strain ( Supplementary Fig. 11 in Supplementary Note 11 ) and lattice distortion ( Supplementary Figs 12 and 13 in Supplementary Note 9 ) and the electrical tunability by gate voltage ( Supplementary Fig. 1 in Supplementary Note 1 ) are also carefully examined, from which we find Dirac physics is quite robust for a single TL film. Magnetic moments can be introduced into this system by magnetic doping, which have been successfully used for topological insulator materials, such as Sb 2 Te 3 family of materials, to realize the QAH effect [39] . Alternatively, one can also exfoliate the TL of (LaO) 2 (SbSe 2 ) 2 and transfer it to ferromagnetic substrate to induce exchange coupling by ferromagnetic proximity [50] . A similar technique has been applied to the graphene systems to observe the anomalous Hall effect [41] , [51] . The electrical tunability of Dirac physics in this system indicates its potential application in various fields. For example, we have shown that a topological phase transition between the QAH states with different quantized Hall conductance can be achieved by controlling electric fields, which will be useful for the experimental study of critical phenomena of topological phase transitions [39] , [52] . Moreover, superconductivity has been realized in (LaO) 2 (BiS 2 ) 2 (refs 21 , 22 , 23 , 26 ) or in LaOFeAs, a well-studied unconventional superconductor with a similar crystal structure [53] . Therefore, it is possible to fabricate heterostructures combining (LaO) 2 (SbSe 2 ) 2 and these superconducting materials, which provide a new flatform to study the coexistence of Dirac physics and superconductivity. Computational methods All the first-principles calculations are based on the density-functional theory as implemented in the Vienna ab initio simulation package [54] , [55] . The projector augmented wave method [56] is used, with a kinetic energy cutoff of 400 eV for the plane wave basis set. The generalized gradient approximation of the Perdew–Burke–Ernzerhof type functional [57] is adopted to describe the exchange-correlation interaction. In the crystal structure, we take the experimental lattice constants: a =4.13 Å and c =14.17 Å (ref. 20 ). For the TL thin film, we build a slab model with a vacuum region of 14 Å to decouple the consecutive slabs in the supercell approach. Γ-centred k -point meshes of dimensions 13 × 13 × 5 and 13 × 13 × 1 are used in the bulk and slab calculations, respectively. The SOC is employed in all electronic structure calculations. We also perform electronic band calculations using the WIEN2K package [58] and reproduce energy dispersion obtained by Vienna ab initio simulation package. The 18 × 18 tight-binding Hamiltonian, which nicely captures the low-energy physics around the Fermi level, is constructed using the maximal localized Wannier function method [44] , [45] . We choose p x , p y , p z states of Sb and Se atoms as the projection centres. How to cite this article: Dong, X.-Y. et al . Electrically tunable multiple Dirac cones in thin films of the (LaO) 2 (SbSe 2 ) 2 family of materials. Nat. Commun. 6:8517 doi: 10.1038/ncomms9517 (2015).